A solid–solid phase transition in carbon dioxide at high pressures and intermediate temperatures Despite its terrestrial abundance and astrochemical significance, many aspects of the phase diagram of solid carbon dioxide remain uncertain or unknown. The observed transition pressures from cubic to orthorhombic phase range widely from 2.5 GPa at 80 K to above 18 GPa at room temperature. The vibrational Raman bands that appear at higher pressure and serve as a decisive proof of the existence of the orthorhombic phase have never been assigned. Here we introduce a general ab initio computational method that can predict the Gibbs free energies and thus phase diagrams of molecular crystals. Using this with second-order Møller—Plesset perturbation theory, we obtain the transition pressure of 13 GPa at 0 K with small temperature dependence, which is in line with many experiments. We also computationally reproduce the vibrational Raman bands and explain the pressure dependence of the structure parameters and Raman band positions of both phases quantitatively. A b initio computational prediction of crystal structures, spectra and phase diagrams has long been a goal of chemists, physicists and materials scientists. The difficulty of such prediction arises from the fact that atoms and molecules in a crystal are bound together by a variety of forces (covalent, ionic, hydrogen-bond and dispersion), whose strengths span three orders of magnitude (100 to 0.1 kJ mol −1 ). This may be compared with the free energy differences of a few kJ mol −1 or less, determining the relative stability of crystalline polymorphs. Density functional theory (DFT), despite its usefulness and improvements in its approximations [1] , has fundamental limitations, two of the severest being the inability to systematically increase its accuracy and the lack of dispersion interactions. Systematic approximations of ab initio molecular orbital theory must be extended to solids. The simplest in this category is the second-order Møller—Plesset perturbation (MP2) method, which can treat all of the aforementioned interactions accurately. However, the computational cost of MP2 is so great that its routine applications to solids are still difficult. This situation is improving rapidly at least for a large and important class of solids known as molecular crystals. Molecular crystals are chemists' solids, so to speak, as their properties can be understood and even controlled by those of the constituent molecules. They include ices of atmospheric species [2] , [3] , drugs [4] , [5] and explosives [6] . They are also related to organic superconductors and other functional materials [7] as well as supramolecular assemblies [8] , [9] . An example in the first category is solid carbon dioxide (CO 2 ), one of nature's most important molecular crystals. Despite its abundance in the Earth's atmosphere and ubiquity in other planets and asteroids in its ice forms, there remain many gaps in our knowledge of the phase diagram of CO 2 [2] , [10] . Today, intense experimental efforts are devoted to explore the high pressure–temperature range in which non-molecular phases [11] , [12] , [13] , [14] , [15] , [16] , [17] , [18] , [19] are observed. The phase diagram in the lower pressure–temperature range is relatively well characterized, yet some aspects of the phases there remain uncertain or unknown to this day. More specifically, when Aoki et al . [20] determined by x-ray diffraction the crystal structure of an orthorhombic (Cmca) phase, the dry ice or the cubic (Pa3) phase (I) had been the only established crystalline phase of CO 2 ( Fig. 1 ). The orthorhombic phase was identified as the high-pressure phase III initially detected by Hanson [21] with Raman spectroscopy. This phase was also responsible for the slight volume collapse occurring at around 12 GPa in the equation-of-state measurement of Liu [22] , who speculated a transition involving the tilting of the molecules. The reported transition pressures at room temperature range widely from 10 GPa (ref. 20 ), 12 GPa (ref. 23 ) to above 18 GPa (ref. 21 ). The transition pressure upon unloading can be as low as somewhere between 4.5 and 2.5 GPa at 80 K (ref. 24 ). There is an extraordinary hysteresis in the transition, obscuring the precise transition pressure and its temperature dependence. 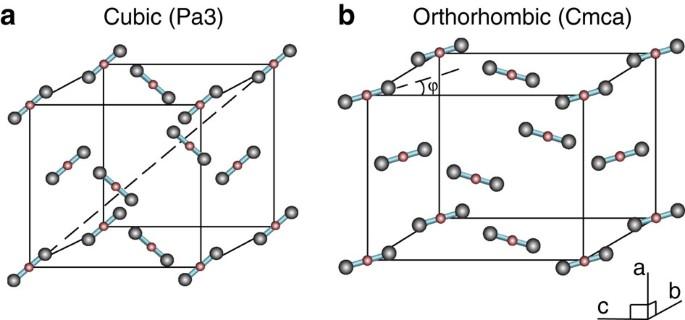Figure 1: Structures of CO2-I and III. The CO2molecules are in the bodydiagonal directions in (a) phase I (Pa3), whereas they are on thebcplanes in (b) phase III (Cmca). Figure 1: Structures of CO 2 -I and III. The CO 2 molecules are in the bodydiagonal directions in ( a ) phase I (Pa3), whereas they are on the bc planes in ( b ) phase III (Cmca). Full size image Interestingly, phase III is reached only by the low-temperature compression of phase I [25] . This implies that phase III is a metastable, kinetically trapped state; there is an underlying phase (II) [17] , [26] , [27] with a lower free energy than phase III. Perhaps the most accurate phase diagram of CO 2 available today is a composite obtained from the experimental data of Litasov et al . [28] , Giordano et al . [29] , [30] and Iota et al . [17] , [25] , which is reproduced in Fig. 2 (the broken line separating phases II and III is a kinetic line). This diagram seems consistent with the observation that, above 400 K, the high-pressure phase transition occurs abruptly at 12–13 GPa, as opposed to sluggishly at lower temperatures. 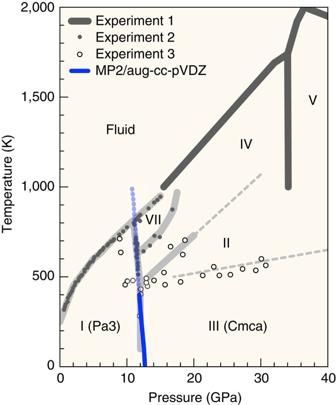Figure 2: Phase diagram. The calculated phase boundary between CO2-I and III is superimposed on the experimentally inferred phase diagram of CO2(data sets 1, 2 and 3 are from Litasovet al.28, Giordanoet al.29,30and Iotaet al.17,25, respectively). The boundary between phases II and III (thin broken line) is a kinetic line. Figure 2: Phase diagram. The calculated phase boundary between CO 2 -I and III is superimposed on the experimentally inferred phase diagram of CO 2 (data sets 1, 2 and 3 are from Litasov et al . [28] , Giordano et al . [29] , [30] and Iota et al . [17] , [25] , respectively). The boundary between phases II and III (thin broken line) is a kinetic line. Full size image The large hysteresis of the phase transition and the metastability of phase III make it difficult to characterize them by experimental means alone; accurate computational assistance is essential. In fact, the high-pressure phase transition from I to III was computationally predicted by Kuchta and Etters [31] , [32] , [33] prior to the x-ray diffraction study [20] . Their calculated value of the CO 2 tilt angle ϕ of 52° was in exact agreement with the observed. Also, the DFT study by Bonev et al . [34] ruled out the experimentally derived hypothesis [12] that phase III was a high-strength material with the bulk modulus of 87 GPa and was not a molecular crystal. These pioneering calculations were, however, not without serious limitations. Those of Kuchta and Etters [31] , [32] , [33] were based on empirical force fields and their predicted transition pressure of 4.3 GPa was too low. The DFT calculations [34] also lacked dispersion interactions, which were shown by us [35] to be crucial cohesive forces in CO 2 -I. Furthermore, despite the fact that Hanson's Raman spectra [21] were the first decisive proof of the existence of phase III, no direct simulation of the spectra supporting this assignment has yet been performed. This article reports an advance in computational machinery [36] , [37] that enables routine ab initio calculations of the free energies of general molecular crystals at finite pressures [38] and temperatures and thus of phase diagrams from first principles. We demonstrate the utility of this method through its application to the structures, equations of state and Raman spectra of both phases I and III of CO 2 as well as the solid–solid phase transition between them. We use MP2 with the exact electronic Hamiltonian (as opposed to empirical or modified Hamiltonians in previous calculations), which is the simplest theory that can describe all cohesive interactions in solid CO 2 simultaneously, accurately and on an equal footing. MP2/aug-cc-pVDZ predicts the transition pressure of 13 GPa (or a few GPa less at a larger basis set) at 0 K with small temperature dependence, which is in line with many experimental reports, while exposing the limitations of the DFT calculation [34] , predicting a higher transition pressure and greater temperature dependence, and of the empirical calculations [31] , [32] , [33] , yielding too low a transition pressure. Equations of state The pressure—volume curves of CO 2 -I and III are drawn in Fig. 3 . In Table 1 , the calculated lattice constants and tilt angle ( ϕ ) at 11.8 GPa are compared with the experimental values [20] and with those obtained with the empirical force field by Kuchta and Etters [31] . Note that in addition to a, b, c, and ϕ , the CO bond lengths in both CO 2 -I and III have also been optimized at each pressure in our calculations, which, therefore, constitute full optimization with only symmetry constraints imposed. 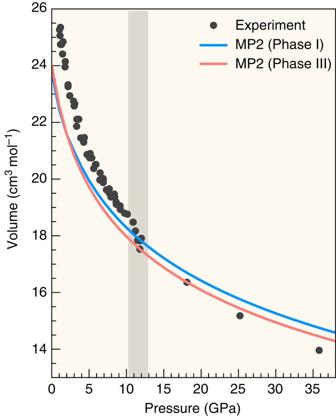Figure 3: Equations of state. The calculated pressure dependence of the volume of CO2-I and III is plotted along with the experimental data from Liu22. The latter seem to exhibit the volume collapse between 10–13 GPa (shaded area) as indication of a solid–solid phase transition. Figure 3: Equations of state. The calculated pressure dependence of the volume of CO 2 -I and III is plotted along with the experimental data from Liu [22] . The latter seem to exhibit the volume collapse between 10–13 GPa (shaded area) as indication of a solid–solid phase transition. Full size image Table 1 Structural parameters of CO 2 -I and III. Full size table For both phases, MP2 with the aug-cc-pVDZ basis set predicts slightly more compact and stiffer solids at lower pressures than experiments [20] , [39] . This may be due to the overestimation of dispersion or quadrupole—quadrupole interactions or both in MP2. With increasing pressure, however, agreement between MP2 and experiments improves and becomes nearly exact (except for c of phase III) at 11.8 GPa, where the x-ray diffraction for CO 2 -III was performed [20] . This trend is commonly observed [38] . The accuracy of the empirical calculation of Kuchta and Etters [31] reported before the x-ray diffraction study is simply astonishing. Both our MP2 calculations and the one by Kuchta and Etters [31] as well as the DFT study of Bonev et al . [34] record ~ 2% volume reduction upon transition from I to III. This volume difference persists (if not grows) with pressure according to both MP2 and DFT calculations. This is consistent with the experimental equation-of-state plot [22] reproduced in Fig. 3 , which shows a visible drop in the volume at about 12 GPa. Given the small temperature dependence of the transition pressure (see below), the driving force of this high-pressure transition may be this small volume reduction. The measured values of volume at pressures greater than 12 GPa tend to fall on the MP2 results of phase III until MP2 again begins to predict slightly too stiff a solid. Overall, the structural data predicted by MP2 are fully consistent with the experimental data. 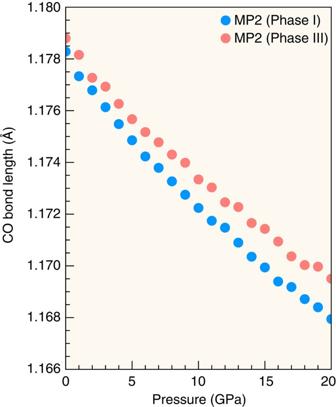Figure 4: CO bond lengths. The pressure dependence of the calculated CO bond lengths of CO2-I and III is plotted. Figure 4 plots the CO bond lengths of both phases as a function of pressure. They decrease nearly linearly with pressure and by roughly 1% upon loading of 20 GPa. Despite the smaller volumes at most pressures, the molecules in phase III are more relaxed with systematically greater bond lengths than in phase I. This is most likely due to the preferable mutual orientations of CO 2 in phase III than in phase I. The differences in CO bond length between the two phases also seem to grow with pressure, which may contribute at least partly to the relative stability of phase III over I at higher pressures. That the intramolecular structural and energy changes as well as intermolecular contributions are taken into account on an equal footing is one of the advantages of ab initio methods. Figure 4: CO bond lengths. The pressure dependence of the calculated CO bond lengths of CO 2 -I and III is plotted. Full size image Vibrational spectra Next, we turn to the spectral data. 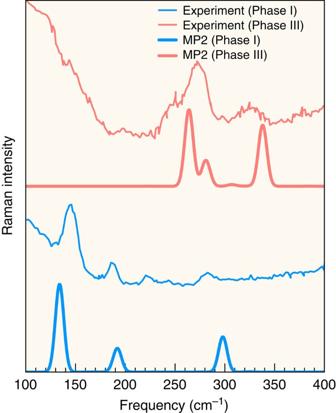Figure 5: Raman spectra. The calculated and observed21Raman spectra of CO2-I (at 14.5 GPa) and III (at 18.0 GPa) are compared in the librational region. The calculated spectra are convoluted with a Gaussian with a full-width half-maximum of 10 cm−1. Figure 5 compares the calculated and observed [21] Raman spectra of CO 2 -I (at 14.5 GPa) and III (at 18.0 GPa). Upon pressure increase, three new Raman bands at 245, 270 and 320 cm −1 appear (top trace), serving as the most decisive proof of the existence of the new phase (III) suggested earlier by the equation-of-state measurement [22] . Our MP2 simulations reproduce the spectra of both phases with remarkable accuracy. CO 2 -I at 14.5 GPa is predicted to display three intense Raman bands in the librational region, which are easily assigned to the three observed bands labelled L 1 , L 2 and L 3 in Fig. 1 of Hanson [21] . CO 2 -III at 18.0 GPa also has three discernible Raman bands in the simulated spectrum, but at rather different frequencies (250–350 cm −1 ), which are again readily assignable to the bands labelled 1, 2 and 3 by Hanson. The agreement in peak positions between theory and experiment is quantitative and the agreement in intensities is also satisfactory. This renders strong computational support for Hanson's assignment [21] of the Raman bands at 18.0 GPa to phase III. Figure 5: Raman spectra. The calculated and observed [21] Raman spectra of CO 2 -I (at 14.5 GPa) and III (at 18.0 GPa) are compared in the librational region. The calculated spectra are convoluted with a Gaussian with a full-width half-maximum of 10 cm −1 . 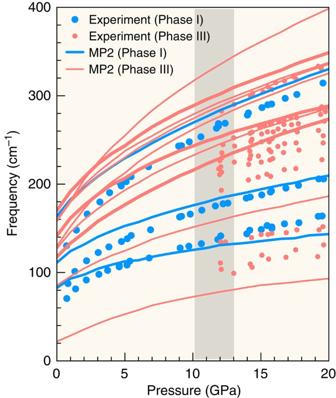Figure 6: Raman band positions. The pressure dependence of the calculated and observed40frequencies of the Raman bands of CO2-I and III is plotted in the librational region. The bold curves in red correspond to the three prominent Raman peaks of CO2-III inFig. 5. Full size image Figure 6 shows the pressure dependence of these and other Raman band positions. While the observed Raman bands due to CO 2 -I (blue circles) are unmistakably identified because of the high symmetry of the crystal, it is not clear which additional observed features (red circles) belong to CO 2 -III above 12 GPa. Nevertheless, MP2 reproduces accurately the observed rates of frequency increase with pressure [40] . Figure 6: Raman band positions. The pressure dependence of the calculated and observed [40] frequencies of the Raman bands of CO 2 -I and III is plotted in the librational region. The bold curves in red correspond to the three prominent Raman peaks of CO 2 -III in Fig. 5 . Full size image Phase diagram Given the accurate structures and phonon density of states (DOS) in the low frequency regions of CO 2 -I and III predicted by MP2, we are in a position to calculate the small salient portion of the phase diagram of CO 2 and the transition pressure as a function of temperature. Our MP2 result of the phase boundary between I and III is superimposed as a blue curve in Fig. 2 . MP2 predicts the transition pressure to be 12.7 GPa at 10 K, which slightly decreases to 12.6 GPa at 100 K, 12.3 GPa at 200 K, 12.1 GPa at 300 K and 11.9 GPa at 400 K. The calculated boundary above this temperature (blue broken line) is probably not meaningful, given the other phases experimentally inferred to exist there. These calculated transition pressures are slightly above the observed range of 10–12 GPa (see the introductory paragraphs). The small temperature dependence, that is, the nearly vertical phase boundary between CO 2 -I and III, is also consistent with the small range of median transition pressures measured at various temperatures between 40 K to room temperature. The DFT calculations by Bonev et al . [34] predict the transition pressures that depend strongly on temperature, going from about 16 GPa at 0 K to about 11 GPa at 350 K, which disagrees with our MP2 results. The experimental data, although not clearcut because of the large hysteresis, seems more in line with MP2 than DFT. Interestingly, DFT predicts [34] a vertical phase boundary at 11 GPa between CO 2 -I and II (P4 2 /mmm). This result should not be taken to indicate that what was believed to be CO 2 -III (Cmca) in many experiments was indeed CO 2 -II (P4 2 /mmm); our MP2 calculations on the structure, spectra and phase boundary are all consistent with the interpretation that phase III is Cmca. 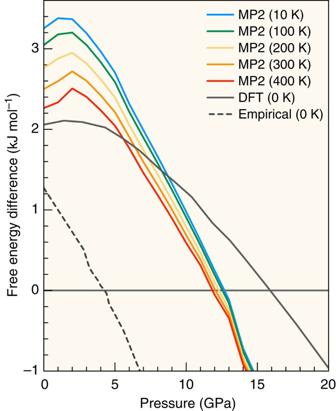Figure 7: Gibbs free energies. The Gibbs free energy differences between CO2-I and III (a positive value means that phase I is more stable) are given as a function of pressure. The solid curves are from second-order Møller—Plesset perturbation calculations (this work) except for the grey curve, which is from the density functional calculations of Bonevet al.34The broken curve is from the empirical-force-field calculations of Kuchta and Etters31. Gibbs free energies Figure 7 shows the free energy differences between phases I and III as a function of pressure and temperature. The general shape of the curves predicted by MP2 is similar to the one from DFT [34] , including the maximum at a few GPa except that the transition pressure predicted by DFT seems too high. With increasing pressure, the effect of temperature diminishes and the five MP2 curves at five different temperatures converge toward one. This is expected and traced to the hardening of acoustic phonons at high pressures. The free energy difference predicted by the empirical force field [31] differs greatly from MP2 or DFT and is likely wrong. Given the success of the empirical force field in predicting the crystal structures, this implies the importance of intramolecular structural changes upon compression (see Fig. 4 ), an effect included in MP2 and DFT, but not in the empirical method. Figure 7: Gibbs free energies. The Gibbs free energy differences between CO 2 -I and III (a positive value means that phase I is more stable) are given as a function of pressure. The solid curves are from second-order Møller—Plesset perturbation calculations (this work) except for the grey curve, which is from the density functional calculations of Bonev et al . [34] The broken curve is from the empirical-force-field calculations of Kuchta and Etters [31] . Full size image The largest source of errors in our calculations is most likely the basis set [41] and its impact is the greatest in the free energy differences. We have, therefore, performed MP2/aug-cc-pVTZ calculations on enthalpy differences between the two phases. The results obtained with the aug-cc-pVTZ basis set are found to be +2.2, −2.1 and −3.5 kJ mol −1 at 0, 14 and 18 GPa (a positive value means that phase I is more stable), which are approximately 1.5 kJ mol −1 lower than the corresponding values (+3.6, −0.5 and −2.0 kJ mol −1 , respectively) obtained with the aug-cc-pVDZ basis set. These suggest that the free energy difference curves shown in Fig. 7 are qualitatively correct, but a basis-set extension stabilizes phase III more than phase I and shifts the I–III transition pressure to a lower value by a few GPa, possibly for better agreement with experiments. Other potentially significant sources of errors are discussed in the Methods section and include higher-order correlation and three-body dispersion effects [42] , [43] . All must be taken into account to reach the so-called ‘chemical accuracy’ [44] of 4 kJ mol −1 in energy differences. We have developed an ab initio electron-correlated method generally applicable to periodic and nonperiodic molecular crystals at finite pressures and temperatures, which, therefore, reports Gibbs free energies and phase diagrams from first principles. It is based on an embedded-fragment approach and can be combined with any electron-correlation theory including but not limited to MP2. Unlike planewave-based methods for crystals, this method can compute phonon dispersion in the entire reciprocal space without a costly supercell approach in addition to the frequencies and intensities of the infrared and Raman-active phonons occurring at the centre of the reciprocal unit cell. It can, therefore, calculate phonon DOS and finite-temperature effects. With this method at the MP2/aug-cc-pVDZ level, we have reproduced quantitatively the frequencies and intensities of the librational Raman bands [21] of both phases I and III using their respective structures, force constants and polarizability derivatives. This supports the original assignments of Hanson [21] . MP2/aug-cc-pVDZ places the transition pressure from phase I to III at 13 GPa at 0 K with small temperature dependence, whereas the basis-set extension to aug-cc-pVTZ lowers the transition pressures by a few GPa, possibly for better agreement with experiments. These are in contrast with the previous DFT study [34] , predicting the transition pressure of 16 GPa at 0 K with much greater temperature dependence. MP2 does not agree with the empirical calculations [31] , the latter proposing a very low transition pressure of 4.3 GPa. The existing body of experimental evidence is more in line with the MP2 results. The ab initio computational method reported here, which can be parallel executed routinely on small computer clusters for infinite three-dimensional solids, therefore, holds exceptional promise in assisting experimental studies of molecular crystals, which are important in high-pressure chemistry [2] , [3] , [6] , solid-state physics [3] , [7] , geochemistry [2] , astrophysics [3] , medicinal chemistry [4] , [5] , supramolecular chemistry [8] , [9] , materials science [4] , [7] and more. Internal energy Our MP2 calculation of the Gibbs free energy of a molecular crystal is based on an embedded-fragment scheme [36] , [37] , [38] , which, in turn, uses the Bethe—Goldstone expansion of the total energy [45] , [46] . The internal energy per unit cell, U e , of solid CO 2 is approximated by where n is a three-integer index of a unit cell, E i ( n ) is, in our case, the MP2/aug-cc-pVDZ energy of the i th CO 2 molecule in the n th unit cell, E i ( 0 ) j ( n ) is the MP2/aug-cc-pVDZ energy of the dimer consisting of the i th molecule in the 0 th unit cell and the j th molecule in the n th unit cell. The prime on the summation symbol indicates that the spurious E i ( 0 ) i ( 0 ) contributions are to be left out of the summation. In this work, the summation over n has been taken in the 3 × 3 × 3 supercell, enclosing 422 dimers. These monomers and dimers are placed in the electrostatic field of the rest of the crystal represented by atomic charges computed by the method developed by Kamiya et al . [47] at the Hartree—Fock (HF) level with the same basis set. These atomic charges are furthermore brought to self consistency with one another [36] . We have taken into account the atomic charges within the 11 × 11 × 11 supercell, consisting of 5,324 molecules. The last term in equation (1), E LR , is the long-range electrostatic contributions and a part of the Madelung constant [37] , [48] . It has been computed with the same atomic charges within the supercell of dimension 41 × 41 × 41, having over a quarter million molecules. Hence, our calculations take into account the 422 most important pairwise electrostatic (that is, induction and hydrogen-bond cooperativity), exchange and correlation (that is, dispersion) interactions at the MP2 level as well as three-body and all higher-order many-body electrostatic interactions within ~20 Å at the HF level. The additional long-range pairwise electrostatic interactions have also been included up to nearly 100 Å or even farther. Enthalpy The effect of pressure has been incorporated [38] by calculating the enthalpy per unit cell, where P is the pressure and V is the unit cell volume, that is, a 3 (phase I) or abc (phase III). Both H e and U e can be analytically differentiated with atomic positions and lattice constants [37] , [38] . With these, we have determined the equilibrium structures and phonon dispersion and DOS of CO 2 -I and III under pressure up to 20.0 GPa. The pressure due to phonons is neglected. We have repeated the single-point enthalpy calculations at the MP2/aug-cc-pVTZ level at 0, 14 and 18 GPa at their respective MP2/aug-cc-pVDZ optimized geometries to assess the effect of a basis-set extension on phase I–III enthalpy differences. Additionally, we have calculated the Raman frequencies and intensities of the zone-centre phonons of CO 2 -I at 14.5 GPa and CO 2 -III at 18.0 GPa using the method developed by He et al . [49] Gibbs free energy The Gibbs free energy per unit cell, G , at temperature T is obtained by evaluating where U v is the zero-point vibrational energy per unit cell at T and S v is the vibrational entropy per unit cell. For a molecular crystal, which has a large band gap, only the temperature effects due to phonons need to be considered. Both U v and S v are derivable from the partition function of phonons, Z v . In the harmonic approximation and atomic units, it is written as [50] , [51] where β=( k B T ) −1 , k B is the Boltzmann constant, and ω n k is the frequency of the phonon in the n th phonon branch with the wave vector k . The latter is determined at the equilibrium structure where H e (not G ) is a minimum. The product over k must be taken over all K evenly spaced grid points of k in the reciprocal unit cell. In this study, the k -grid of 21 × 21 × 21 has been used ( K =9,261). According to thermodynamics [50] , [51] , we have The right-hand sides of these equations can be readily evaluated with phonon dispersion, {ω n k }. The availability of the latter in the entire reciprocal space (not just at the Γ point) is one of the unique advantages of the fragment schemes unconstrained by the periodic boundary conditions. Computer implementation The calculations have been performed by our in-house parallel execution programme, running monomer and dimer MP2 calculations using unmodified Gaussian09 [52] . The structural optimization, vibrational analyses and free energy calculations have been performed with our in-house software. Known limitations Although this constitutes a state-of-the-art calculation for solids and a significant improvement over DFT or empirical calculations, it has numerous sources of errors. The gravest is the approximate nature of MP2 and the incompleteness of the basis sets [41] , [44] . The use of the harmonic approximation in the treatment of phonons is responsible for errors at higher temperatures [49] . Another source of errors is the use of HF in determining the embedding field and its truncation at a finite distance. It also neglects three-body and higher many-body exchange and correlation interactions, which have been shown [42] , [43] to be non-negligible for CO 2 . The agreement between experiment and simulation in this study, therefore, implicitly exploits the cancellation of these errors between two similar structures or phases. However, it should be emphasized that, thanks to the systematic nature of the ab initio molecular orbital theory and embedded-fragment scheme, all of these errors can, in principle, be arbitrarily reduced at an increased computational cost. How to cite this article: Li, J. et al . A solid–solid phase transition in carbon dioxide at high pressures and intermediate temperatures. Nat. Commun. 4:2647 doi: 10.1038/ncomms3647 (2013).